A population of glomerular glutamatergic neurons controls sensory information transfer in the mouse olfactory bulb In sensory systems, peripheral organs convey sensory inputs to relay networks where information is shaped by local microcircuits before being transmitted to cortical areas. In the olfactory system, odorants evoke specific patterns of sensory neuron activity that are transmitted to output neurons in olfactory bulb (OB) glomeruli. How sensory information is transferred and shaped at this level remains still unclear. Here we employ mouse genetics, 2-photon microscopy, electrophysiology and optogenetics, to identify a novel population of glutamatergic neurons (VGLUT3 + ) in the glomerular layer of the adult mouse OB as well as several of their synaptic targets. Both peripheral and serotoninergic inputs control VGLUT3 + neurons firing. Furthermore, we show that VGLUT3 + neuron photostimulation in vivo strongly suppresses both spontaneous and odour-evoked firing of bulbar output neurons. In conclusion, we identify and characterize here a microcircuit controlling the transfer of sensory information at an early stage of the olfactory pathway. In mammals, olfactory sensory neurons project their axons in a receptor-specific manner onto olfactory bulb (OB) glomeruli [1] , [2] . At this level, OSNs establish synaptic contacts with the apical dendrites of OB output neurons and with different populations of juxtaglomerular (JG) cells. Olfactory information is then transferred to olfactory cortices through M/T cells’ axonal projections. JG cells establish dendrodendritic synapses with each other and with M/T cells. Among the various JG cells, a population of excitatory neurons called external tufted (ET) cells, may play a major role in modulating the input from OSNs to M/T cells [3] , [4] , [5] , [6] . The current model describes the transfer of olfactory information as a multistep excitation mechanism (that is, feedforward excitation) in which the inputs to M/T cells is augmented by ET cells. ET cells in fact receive stronger OSN inputs than MCs and are thought to drive OB output neurons through direct glutamatergic synaptic transmission [3] , [4] , [5] , [6] . This feedforward pathway is thought to be extremely important since direct inputs from OSNs to M/T cells are often too weak to evoke action potentials [6] . For this reason, ET cells may represent a critical node to transfer odorant information to cortical areas. Here, we aimed to obtain a molecular marker of ET cells involving vesicular glutamate transporters (VGLUTs) to study how odorant information is transferred in the OB in vivo . VGLUTs are essential to fill glutamate into synaptic vesicles and are sufficient to confer the glutamatergic phenotype [7] , [8] . In mammals, three transporters have been identified: VGLUT1 (also called SLC17A7 (refs 7 , 8 )), VGLUT2 (SLC17A6 (refs 9 , 10 , 11 , 12 )) and VGLUT3 (SLC17A8 (refs 13 , 14 , 15 , 16 )). In the adult OB, M/T cells express VGLUT1 while VGLUT2 is strongly expressed by OSNs terminals [17] , [18] , [19] . In the glomerular layer (GL), unidentified JG cells express VGLUT2 and VGLUT3, some of them being putative ET cells [13] , [19] . In this study, combining mouse genetics, immunohistochemistry and electrophysiology, we describe a previously uncharacterized population of cells expressing VGLUT3. These neurons could be classified as ET cells from a morphological and electrophysiological point of view. However, using optogenetic circuit dissection, we show that VGLUT3 neurons have a different connectivity profile than previously described ET cells and that they differentially connect JG cells and output neurons. Finally, we show that channelrhodopsin stimulation of VGLUT3 neurons strongly suppresses both spontaneous and odour-evoked firing of OB output neurons in vivo . Our data strongly suggest that VGLUT3 neurons can modulate M/T cells firing and as a consequence control the transfer of olfactory information to olfactory cortices. VGLUT3 is expressed by some JG neurons To characterize VGLUT3 neurons of the main OB, we used Vglut3-TOM and Vglut3-ChR2 mice (see Methods and Fig. 1a ). In the OB of adult animals, reporter-expressing neurons were exclusively found in the [13] , [19] GL and displayed the morphology of ET cells characterized by a pear-shaped soma and an apical dendrite ramifying a large portion of a single glomerulus ( Fig. 1b–g ). The labelling was local with no sign of long-range centrifugal projections ( Fig. 1b,c ). VGLUT3 neurons often had axons ramifying into GL, external plexiform layer (EPL), internal plexiform layer and to a lesser extent to the granule cell (GC) layer ( Fig. 1c,d ). 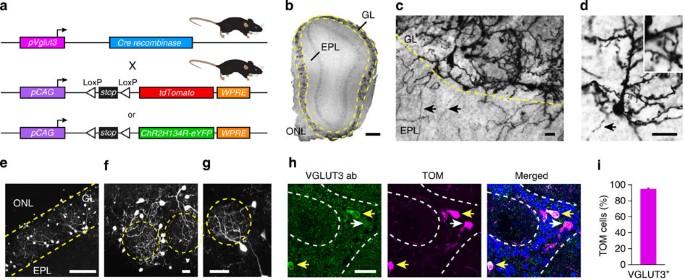Figure 1: VGLUT3 expression defines a neuronal population located in the GL of the mouse OB. (a) Schema of the breeding strategy. A transgenic mouse expressing Cre recombinase under theVglut3promoter (pVglut3) was crossed with two reporter lines conditionally expressing either tdTomato or Channelrhodopsin2-YFP. pCAG:CAGpromoter,WPRE: Woodchuck hepatitis post-transcriptional regulatory element,LoxP: sequence recognized by the Cre recombinase for recombination. (b–d) Coronal sections of the adult OB immunostained for YFP in Vglut3-ChR2 mice. Positive cell bodies were found exclusively in the GL (b, GL, left image). Stained cells often exhibited axons (black arrows,c,d) and spiny dendrites (d). (e–g) Z-stack projections of TOM+neurons imaged in the GL using 2-photon microscopy in 300-μm thick slices of a Vglut3-TOM mouse. The dendritic tuft of TOM+cells extensively arborized individual glomeruli (circular dotted lines inf,g). Some cells had longer dendrites than others (g). ONL: olfactory nerve layer. (h) Antibody staining for VGLUT3 on Vglut3-TOM slices (VGLUT3 ab). Arrows highlight TOM+neurons expressing VGLUT3 (yellow) or not (white). (i) Percentage of TOM+cells stained by the VGLUT3 antibody in 2-month-old animals (n=4 mice, data are shown as mean±s.e.m). Scale bars, 0.3 mm (b), 0.1 mm (e) and 20 μm (c,d,f–h). Figure 1: VGLUT3 expression defines a neuronal population located in the GL of the mouse OB. ( a ) Schema of the breeding strategy. A transgenic mouse expressing Cre recombinase under the Vglut3 promoter ( pVglut3 ) was crossed with two reporter lines conditionally expressing either tdTomato or Channelrhodopsin2-YFP. pCAG: CAG promoter, WPRE : Woodchuck hepatitis post-transcriptional regulatory element, LoxP : sequence recognized by the Cre recombinase for recombination. ( b – d ) Coronal sections of the adult OB immunostained for YFP in Vglut3-ChR2 mice. Positive cell bodies were found exclusively in the GL ( b , GL, left image). Stained cells often exhibited axons (black arrows, c , d ) and spiny dendrites ( d ). ( e – g ) Z-stack projections of TOM + neurons imaged in the GL using 2-photon microscopy in 300-μm thick slices of a Vglut3-TOM mouse. The dendritic tuft of TOM + cells extensively arborized individual glomeruli (circular dotted lines in f , g ). Some cells had longer dendrites than others ( g ). ONL: olfactory nerve layer. ( h ) Antibody staining for VGLUT3 on Vglut3-TOM slices (VGLUT3 ab). Arrows highlight TOM + neurons expressing VGLUT3 (yellow) or not (white). ( i ) Percentage of TOM + cells stained by the VGLUT3 antibody in 2-month-old animals ( n =4 mice, data are shown as mean±s.e.m). Scale bars, 0.3 mm ( b ), 0.1 mm ( e ) and 20 μm ( c , d , f – h ). Full size image To determine whether genetic labelling accurately reported endogenous expression of VGLUT3, we performed immunolabelling for VGLUT3 on slices from 8-week-old Vglut3-TOM mice ( Fig. 1h ). All immunostained VGLUT3 cells were TOM + and ~95% of TOM + cells expressed VGLUT3 (95±1.3%, Fig. 1i ). The remaining fraction may represent either cells starting to express VGLUT3, lack of uniform penetration of the antibody, cells which transiently expressed VGLUT3 or a non-specific expression of the reporter. In summary, Vglut3-reporter mice specifically label glutamatergic neurons in the GL having the morphology of putative ET cells. Heterogeneity of the VGLUT3 population To characterize the glutamatergic neurons located in the GL, we performed immunostaining for VGLUT1 and VGLUT2 on Vglut3-TOM slices from 8-week-old mice ( Fig. 2a and Supplementary Fig. 1a–c ). VGLUT1 + and VGLUT2 + cells were found in the GL, although VGLUT1-expressing cells were more often located at the base of GL (that is, border between GL and EPL). As the expression of VGLUTs may be developmentally regulated, we quantified the density of neurons expressing different VGLUTs in the GL at three postnatal ages (2, 4 and 8 weeks). For all ages, TOM + neurons were three to six times less numerous than VGLUT1 or VGLUT2 neurons ( Fig. 2b–d ). In addition, the number of TOM + cells increased with age ( Fig. 2d ). The average density of TOM + cells was comparable with the density of immunostained VGLUT3 + neurons (average density at 8 weeks=15.8±0.3 × 10 3 mm −3 and 17.5±0.8 × 10 3 mm −3 for VGLUT3 + and TOM + , respectively; unpaired t -test P =0.13, t (3)=1.9, n =4 animals, Fig. 2d ). 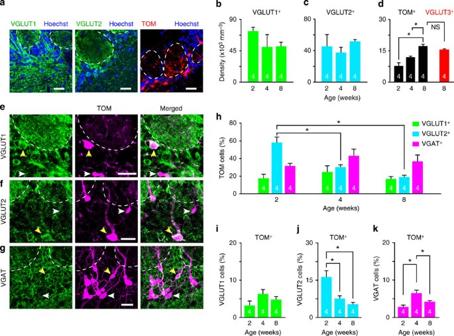Figure 2: Vesicular glutamate and GABA transporters define different subpopulations of VGLUT3 neurons. (a) Confocal images of the GL in OB slices taken from Vglut3-TOM mice and immunostained for VGLUT1 or VGLUT2. Glomeruli boundaries (dotted lines) were visualized by Hoechst staining. (b–d) Age-dependent variation in density of neurons expressing different vesicular transporters in the GL (Kruskal–Wallis ANOVA H(2,12)=3.5,P=0.17 for VGLUT1+and one-way ANOVA F(2,9)=1.35,P=0.3; F(2,9)=0.55,P=0.59; F(2,9)=10.74,P=0.004 for, VGLUT2+and TOM+, respectively).Post hocFischer least significant difference (LSD) test ind: 2 versus 4 weeksP=0.06, 2 versus 8 weeks *P=0.002, 4 versus 8 weeks *P=0.04. TOM+and VGLUT3+density was not statistically different (unpairedt-testt(1.9),P=0.13). (e–g) Confocal images showing co-localization (yellow arrows) and no co-localization (white arrows) of TOM with VGLUT1 (e), VGLUT2 (f) or VGAT (g). (h) Percentage of TOM+cells expressing VGLUT1, VGLUT2 or VGAT (one-way ANOVA F(2,9)=0.67,P=0.53; F(2,9)=26.3,P=2.10−4; F(2,9)=0.91,P=0.44 for VGLUT1+, VGLUT2+and VGAT+, respectively). LSD test for VGLUT2+: 2 versus 4 weeks *P=7.10−4, 2 versus 8 weeks *P=6.10−5, 4 versus 8 weeksP=0.07. (i–k) Percentage of VGLUT1+(i), VGLUT2+(j) or VGAT+(k) cells co-localized with TOM (one-way ANOVA F(2,9)=2.1,P=0.18; F(2,9)=12.5, *P=0.003; F(2,9)=14.4, *P=0.005 for VGLUT1/TOM, VGLUT2/TOM, respectively and Kruskal–Wallis ANOVA H(2,12)=8.8,P=0.013 for VGAT/TOM). LSD test inj:2 versus 4 weeks *P=0.005, 2 versus 8 weeks *P=0.001, 4 versus 8 weeksP=0.35; Kruskal–Wallis test ink: 2 versus 4 weeks *P=0.01, 2 versus 8 weeksP=0.71, 4 versus 8 weeksP=0.23. Data are presented as mean±s.e.m. (white numbers on histograms indicate number of mice). Scale bars, 20 μm. Figure 2: Vesicular glutamate and GABA transporters define different subpopulations of VGLUT3 neurons. ( a ) Confocal images of the GL in OB slices taken from Vglut3-TOM mice and immunostained for VGLUT1 or VGLUT2. Glomeruli boundaries (dotted lines) were visualized by Hoechst staining. ( b – d ) Age-dependent variation in density of neurons expressing different vesicular transporters in the GL (Kruskal–Wallis ANOVA H (2,12) =3.5, P =0.17 for VGLUT1 + and one-way ANOVA F (2,9) =1.35, P =0.3; F (2,9) =0.55, P =0.59; F (2,9) =10.74, P =0.004 for, VGLUT2 + and TOM + , respectively). Post hoc Fischer least significant difference (LSD) test in d : 2 versus 4 weeks P =0.06, 2 versus 8 weeks * P =0.002, 4 versus 8 weeks * P =0.04. TOM + and VGLUT3 + density was not statistically different (unpaired t -test t (1.9), P =0.13). ( e – g ) Confocal images showing co-localization (yellow arrows) and no co-localization (white arrows) of TOM with VGLUT1 ( e ), VGLUT2 ( f ) or VGAT ( g ). ( h ) Percentage of TOM + cells expressing VGLUT1, VGLUT2 or VGAT (one-way ANOVA F (2,9) =0.67, P =0.53; F (2,9) =26.3, P =2.10 −4 ; F (2,9) =0.91, P =0.44 for VGLUT1 + , VGLUT2 + and VGAT + , respectively). LSD test for VGLUT2 + : 2 versus 4 weeks * P =7.10 −4 , 2 versus 8 weeks * P =6.10 −5 , 4 versus 8 weeks P =0.07. ( i – k ) Percentage of VGLUT1 + ( i ), VGLUT2 + ( j ) or VGAT + ( k ) cells co-localized with TOM (one-way ANOVA F (2,9) =2.1, P =0.18; F (2,9) =12.5, * P =0.003; F (2,9) =14.4, * P =0.005 for VGLUT1/TOM, VGLUT2/TOM, respectively and Kruskal–Wallis ANOVA H (2,12) =8.8, P =0.013 for VGAT/TOM). LSD test in j: 2 versus 4 weeks * P =0.005, 2 versus 8 weeks * P =0.001, 4 versus 8 weeks P =0.35; Kruskal–Wallis test in k : 2 versus 4 weeks * P =0.01, 2 versus 8 weeks P =0.71, 4 versus 8 weeks P =0.23. Data are presented as mean±s.e.m. (white numbers on histograms indicate number of mice). Scale bars, 20 μm. Full size image We then tested whether Vglut3-TOM neurons expressed additional vesicular transporters ( Fig. 2e–g ). Approximately 20% of TOM + neurons co-expressed VGLUT1 independently of age ( Fig. 2h ). In contrast, VGLUT2 co-expression was age dependent, starting at ~60% of the TOM population at 2 weeks and decreasing to ~20% at 8 weeks ( Fig. 2h ). Surprisingly, ~30–40% of TOM + cells co-expressed the vesicular GABA transporter VGAT at all ages ( Fig. 2g,h ). Although some VGLUT3 neurons express additional vesicular transporters, these neurons represent a minor fraction (~5% at 8-week-old age) of the entire VGLUT1 + , VGLUT2 + or VGAT + populations ( Fig. 2i–k ). The expression of different vesicular transporters with VGLUT3 may indicate the existence of different subpopulations of VGLUT3 neurons. To test this possibility, we measured the soma size and observed that different populations of glutamatergic neurons located in the GL could be distinguished. VGLUT1 neurons had larger somata ( Fig. 3a–d ) and may represent tufted cells (TCs) [18] , [19] . In contrast, TOM + and VGLUT2 + cells could not be easily distinguished from each other but had larger soma than GABAergic neurons identified by the expression of the vesicular GABA transporter (VGAT; Fig. 3a–d ). Finally, VGLUT1 + /TOM + , VGLUT2 + /TOM + , VGAT + /TOM + neurons could be distinguished by their soma size and could therefore represent three different subpopulations of VGLUT3 neurons ( Fig. 3e–h ). 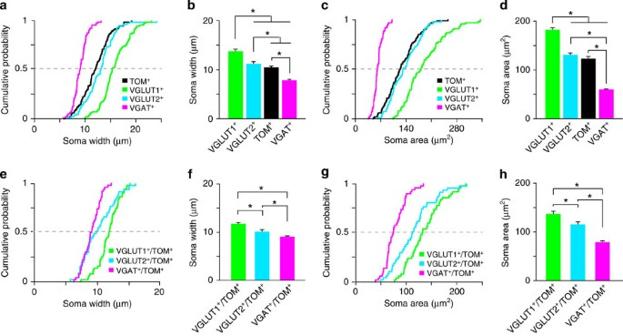Figure 3: Different populations of glutamatergic neurons in the glomerular area differ in soma size. (a) Cumulative distribution (~n=100 cells taken from 5–6 slices from four animals) of soma width measured in different cell populations. All distributions except TOM+versus VGLUT2+are significantly different (Kolmogorov–Smirnov KS testP<0.001). (b) Average soma size measured in different populations of neurons. One-way ANOVA F(3,387)=120.6,P<10−8,:post hocLSD test: VGLUT1 versus VGLUT2 *P=8.1 × 10−15, VGLUT3 versus VGLUT1 *P=2.8 × 10−23, VGLUT3 versus VGLUT2 *P=0.01, VGAT versus VGLUT1 *P=9.5 × 10−57, VGAT versus VGLUT2 *P=8.2 × 10−23, VGAT versus VGLUT3 *P=2.5 × 10−15. (c) Cumulative distribution of soma area in the same populations of neurons. All distributions except TOM+versus VGLUT2+are significantly different (KS testP<0.001). (d) Average soma area measured in different population of neurons. One-way ANOVA F(3,387)=15,P<10−8,post hocLSD test: VGLUT2 versus VGLUT1 *P=3.4 × 10−17, VGLUT3 versus VGLUT1 *P=6.1 × 10−22, VGLUT3 versus VGLUT2P=0.2, VGAT versus VGLUT1 *P=1.10−57, VGAT versus VGLUT2 *P=2.4 × 10−29, VGAT versus VGLUT3 *P=4.2 × 10−25. (e) Cumulative distribution of soma width measured in different subpopulations of TOM+neurons co-expressing different vesicular transporters (n=50 cells taken from 5–6 slices from four animals). All distributions are significantly different (KS test at leastP<0.001). (f) Average soma width measured in different populations of neurons. One-way ANOVA F(2,138)=21.4, *P=7.8 × 10−9.Post hocFischer LSD test: VGLUT2/TOM versus VGLUT1/TOM *P=1.1 × 10−4, VGAT/TOM versus VGLUT1/TOM *P=1.4 × 10−9, VGAT/TOM versus VGLUT2/TOM *P=0.01. (g) Cumulative distribution of soma area in the same populations of neurons. All distributions are significantly different (KS testP<0.001). (h) Average soma area measured in different populations of neurons. One-way ANOVA F(2,138)=35.3, P=4.10−13. LSD test at least *P=0.002. VGLUT2/TOM versus VGLUT1/TOM *P=0.002, VGAT/TOM versus VGLUT1/TOM *P=7.3 × 10−14, VGAT/TOM versus VGLUT2/TOM *P=7.1 × 10−7. Figure 3: Different populations of glutamatergic neurons in the glomerular area differ in soma size. ( a ) Cumulative distribution (~ n =100 cells taken from 5–6 slices from four animals) of soma width measured in different cell populations. All distributions except TOM + versus VGLUT2 + are significantly different (Kolmogorov–Smirnov KS test P <0.001). ( b ) Average soma size measured in different populations of neurons. One-way ANOVA F (3,387) =120.6, P <10 −8 ,: post hoc LSD test: VGLUT1 versus VGLUT2 * P =8.1 × 10 −15 , VGLUT3 versus VGLUT1 * P =2.8 × 10 −23 , VGLUT3 versus VGLUT2 * P =0.01, VGAT versus VGLUT1 * P =9.5 × 10 −57 , VGAT versus VGLUT2 * P =8.2 × 10 −23 , VGAT versus VGLUT3 * P =2.5 × 10 −15 . ( c ) Cumulative distribution of soma area in the same populations of neurons. All distributions except TOM + versus VGLUT2 + are significantly different (KS test P <0.001). ( d ) Average soma area measured in different population of neurons. One-way ANOVA F (3,387) =15, P <10 −8 , post hoc LSD test: VGLUT2 versus VGLUT1 * P =3.4 × 10 −17 , VGLUT3 versus VGLUT1 * P =6.1 × 10 −22 , VGLUT3 versus VGLUT2 P =0.2, VGAT versus VGLUT1 * P =1.10 −57 , VGAT versus VGLUT2 * P =2.4 × 10 −29 , VGAT versus VGLUT3 * P =4.2 × 10 −25 . ( e ) Cumulative distribution of soma width measured in different subpopulations of TOM + neurons co-expressing different vesicular transporters ( n =50 cells taken from 5–6 slices from four animals). All distributions are significantly different (KS test at least P <0.001). ( f ) Average soma width measured in different populations of neurons. One-way ANOVA F (2,138) =21.4, * P =7.8 × 10 −9 . Post hoc Fischer LSD test: VGLUT2/TOM versus VGLUT1/TOM * P =1.1 × 10 −4 , VGAT/TOM versus VGLUT1/TOM * P =1.4 × 10 −9 , VGAT/TOM versus VGLUT2/TOM * P =0.01. ( g ) Cumulative distribution of soma area in the same populations of neurons. All distributions are significantly different (KS test P <0.001). ( h ) Average soma area measured in different populations of neurons. One-way ANOVA F (2,138) =35.3, P =4.10 −13 . LSD test at least * P =0.002. VGLUT2/TOM versus VGLUT1/TOM * P =0.002, VGAT/TOM versus VGLUT1/TOM * P =7.3 × 10 −14 , VGAT/TOM versus VGLUT2/TOM * P =7.1 × 10 −7 . Full size image Our data suggest that a subpopulation of Vglut3-TOM neurons may not only be glutamatergic but may also have a GABAergic phenotype, as indicated by the expression of the vesicular GABA transporter. In agreement, some VGLUT3 neurons, but not VGLUT1 and VGLUT2 cells, expressed the GABA synthetizing enzyme GAD67 suggesting that co-expression of GABAergic markers is unique to the VGLUT3 population in the GL of the mouse OB ( Fig. 4a–d ). We then tested whether the GABAergic subpopulation of Vglut3-TOM neurons expressed known markers for GABAergic periglomerular cells, such as the Ca 2+ binding proteins calretinin (CALR) and calbindin (CALB) [20] or the tyrosine hydroxylase (TH) enzyme [21] . TOM + neurons frequently expressed CALB but rarely calretinin or TH ( Fig. 5a–c ). While most GABAergic Vglut3-TOM neurons expressed CALB (94±2.9%, n =4 mice), ~70% of the VGLUT3 + /CALB + neurons were found to be GAD67 positive ( Fig. 5d ), suggesting that some CALB + neurons are exclusively glutamatergic. 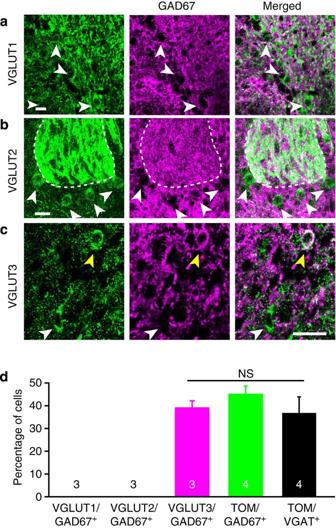Figure 4: Neurons expressing VGLUT3 are the only glutamatergic neurons of the GL exhibiting a GABAergic phenotype. (a–c) Confocal images acquired from the GL of 2-month-old C57BL/6J mice double stained for VGLUT1 and GAD67 (a), VGLUT2 and GAD67 (b) VGLUT3 and GAD67 (c). Yellow and white arrows indicate co-stained and not co-stained cells, respectively. Scale bars, 20 μm. (d) Percentage of VGLUT1+, VGLUT2+and VGLUT3+cells expressing GAD67. Note that the percentage of TOM+/GAD67+and TOM+/VGAT+neurons was not statistically different from VGLUT3+/GAD67+-expressing cells. One-way ANOVA F(3,11)=0.6,P=0.5. Data are presented as mean±s.e.m. Numbers on histograms indicate number of mice. Figure 4: Neurons expressing VGLUT3 are the only glutamatergic neurons of the GL exhibiting a GABAergic phenotype. ( a – c ) Confocal images acquired from the GL of 2-month-old C57BL/6J mice double stained for VGLUT1 and GAD67 ( a ), VGLUT2 and GAD67 ( b ) VGLUT3 and GAD67 ( c ). Yellow and white arrows indicate co-stained and not co-stained cells, respectively. Scale bars, 20 μm. ( d ) Percentage of VGLUT1 + , VGLUT2 + and VGLUT3 + cells expressing GAD67. Note that the percentage of TOM + /GAD67 + and TOM + /VGAT + neurons was not statistically different from VGLUT3 + /GAD67 + -expressing cells. One-way ANOVA F (3,11) =0.6, P =0.5. Data are presented as mean±s.e.m. Numbers on histograms indicate number of mice. 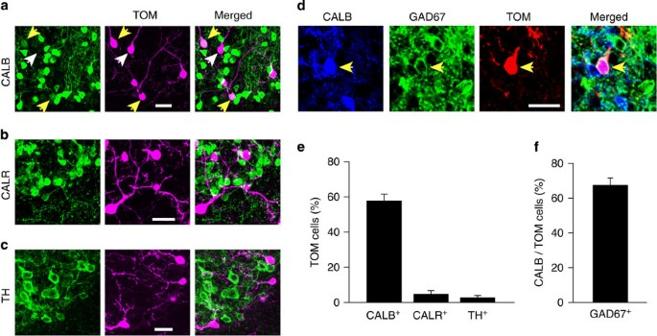Figure 5: Immunohistochemical characterization of GABAergic VGLUT3 neurons. (a–c) Confocal images acquired from the GL of OB slices taken from Vglut3-TOM mice and immunostained for calbindin (CALB,a), calretinin (CALR,b) or tyrosine hydroxylase (TH,c). Arrows point to TOM+cells co-expressing (yellow) or not co-expressing (white) the tested marker. (d) Confocal images showing a TOM+cell co-expressing CALB and GAD67 (yellow arrow). (e) Percentage of TOM+cells expressing CALB, CALR or TH (n=4, 8-week-old mice in each group; quantifications were done for each animal on ~100 cells imaged from ~6 slices). (f) Percentage of CALB/TOM cells expressing GAD67. Data are presented as mean±s.e.m. Scale bars, 20 μm. Full size image Figure 5: Immunohistochemical characterization of GABAergic VGLUT3 neurons. ( a – c ) Confocal images acquired from the GL of OB slices taken from Vglut3-TOM mice and immunostained for calbindin (CALB, a ), calretinin (CALR, b ) or tyrosine hydroxylase (TH, c ). Arrows point to TOM + cells co-expressing (yellow) or not co-expressing (white) the tested marker. ( d ) Confocal images showing a TOM + cell co-expressing CALB and GAD67 (yellow arrow). ( e ) Percentage of TOM + cells expressing CALB, CALR or TH ( n =4, 8-week-old mice in each group; quantifications were done for each animal on ~100 cells imaged from ~6 slices). ( f ) Percentage of CALB/TOM cells expressing GAD67. Data are presented as mean±s.e.m. Scale bars, 20 μm. Full size image In summary, Vglut3-TOM cells represent a heterogeneous population of JG neurons co-expressing different glutamate and GABA vesicular transporters. Electrophysiological properties of VGLUT3 neurons Since VGLUT3 neurons had the morphology of putative ET cells, we tested whether they displayed the electrophysiological properties previously reported for such neurons: (1) low membrane resistance; (2) resting membrane potential around −50 mV; (3) presence of sag and rebound spiking in response to hyperpolarizing current injection reflecting the activation of a hyperpolarization-activated cation current (I h ); and (4) spontaneous rhythmic activity persisting in presence of GABAergic and glutamatergic receptor antagonists [22] , [23] . To account for the diversity of the VGLUT3 population, we recorded a large number of cells with different soma sizes and location in the GL. All VGLUT3 neurons exhibited a unique apical dendrite arborizing a single glomerulus and axons running in the GL/EPL, sometimes reaching the granule cell layer ( Fig. 6a–e ). In agreement with the diversity of ET cells previously reported [22] , [23] , [24] , [25] , [26] , [27] , [28] , several cells had basal dendrites whereas other did not. 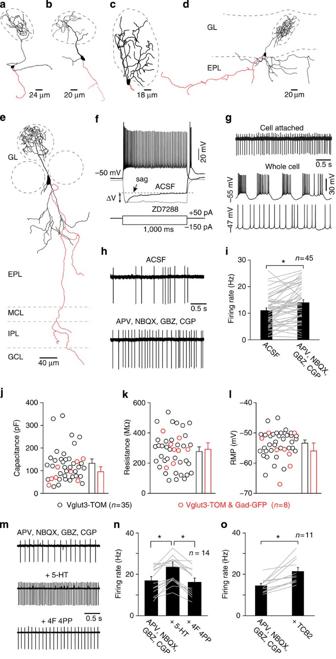Figure 6: Vglut3 neurons exhibit electrophysiological properties of ET cells. (a–e) Morphology of Vglut3-TOM neurons patched and filled with biocytin (axons in red). GCL: granule cell layer, IPL: internal plexiform layer. (f) Typical response of a TOM+neuron to the injection of current pulses. Note the presence of sag (blocked by the specific Ihcurrent antagonist ZD7288 10 μM) and rebound spiking following hyperpolarization. ΔV: voltage difference between beginning and end of sag. (g) Spontaneous firing activity recorded from a TOM+neuron. Note the firing behaviour depended on the resting membrane potential. (h) Vglut3-TOM neurons spontaneously fire in the presence of 100 dl-APV, 10 NBQX, 10 SR-95531 (GBZ), 10 CGP 35348 (in μM, antagonists mix). (i) Summary graph showing the average firing frequency computed for different cells (from 45 slices from 25 animals) before and during drug application (grey lines: individual cell;n=45, Wilcoxon matched pairs test *P=0.0003,Z(44)=3.65). (j–l) Summary graphs showing single cells’ value and average for Vglut3-TOM (cells recorded in nine mice) and Vglut3-TOM/Gad67-GFP neurons (cells recorded in two mice) for capacitance (j, Mann–WhitneyU-testP=0.77,Z(41)=−0.3), membrane resistance (k, Mann–WhitneyU-testP=0.22,Z(41)=1.23), resting membrane potential (l; RMP, Mann–WhitneyU-testP=0.35,Z(41)=0.94). (m) Spontaneous firing activity recorded from a TOM+neuron before and after sequential application of 40 μM 5-HT and the 5-HT2A receptor antagonist 4F-4PP (5 μM). (n–o) Summary graphs showing the average firing frequency computed for each cell (grey lines) or the population (black bars) during different drug conditions (n, one-way repeated measures ANOVA F(2,26)=24.1,P=1.3 × 10−6;post hocFischer LSD test: drugs versus 5-HT *P=10−7,t(26)=5.5; 5-HT versus 4F-4PP *P=8.3 × 10−7,t(26)=6.4; drugs versus 4F-4PPP=0.35,t(26)=0.95). Application of 5-HT2A receptor agonist TCB-2 (10 μM) increased the firing frequency (o, Wilcoxon matched pairs testP=0.0014,Z=3.2). All data are presented as mean±s.e.m. Figure 6: Vglut3 neurons exhibit electrophysiological properties of ET cells. ( a – e ) Morphology of Vglut3-TOM neurons patched and filled with biocytin (axons in red). GCL: granule cell layer, IPL: internal plexiform layer. ( f ) Typical response of a TOM + neuron to the injection of current pulses. Note the presence of sag (blocked by the specific I h current antagonist ZD7288 10 μM) and rebound spiking following hyperpolarization. ΔV: voltage difference between beginning and end of sag. ( g ) Spontaneous firing activity recorded from a TOM + neuron. Note the firing behaviour depended on the resting membrane potential. ( h ) Vglut3-TOM neurons spontaneously fire in the presence of 100 dl-APV, 10 NBQX, 10 SR-95531 (GBZ), 10 CGP 35348 (in μM, antagonists mix). ( i ) Summary graph showing the average firing frequency computed for different cells (from 45 slices from 25 animals) before and during drug application (grey lines: individual cell; n =45, Wilcoxon matched pairs test * P =0.0003, Z (44)=3.65). ( j – l ) Summary graphs showing single cells’ value and average for Vglut3-TOM (cells recorded in nine mice) and Vglut3-TOM/Gad67-GFP neurons (cells recorded in two mice) for capacitance ( j , Mann–Whitney U -test P =0.77, Z (41)=−0.3), membrane resistance ( k , Mann–Whitney U -test P =0.22, Z (41)=1.23), resting membrane potential ( l ; RMP, Mann–Whitney U -test P =0.35, Z (41)=0.94). ( m ) Spontaneous firing activity recorded from a TOM + neuron before and after sequential application of 40 μM 5-HT and the 5-HT2A receptor antagonist 4F-4PP (5 μM). ( n – o ) Summary graphs showing the average firing frequency computed for each cell (grey lines) or the population (black bars) during different drug conditions ( n , one-way repeated measures ANOVA F (2,26) =24.1, P =1.3 × 10 −6 ; post hoc Fischer LSD test: drugs versus 5-HT * P =10 −7 , t (26)=5.5; 5-HT versus 4F-4PP * P =8.3 × 10 −7 , t (26)=6.4; drugs versus 4F-4PP P =0.35, t (26)=0.95). Application of 5-HT2A receptor agonist TCB-2 (10 μM) increased the firing frequency ( o , Wilcoxon matched pairs test P =0.0014, Z =3.2). All data are presented as mean±s.e.m. Full size image During whole-cell recording, we injected hyperpolarizing steps of current while holding the membrane potential at ~−50 mV. All tested cells ( n =50) had sag blocked by the specific I h antagonist ZD7288 ( Fig. 6f ; ΔV=16.1±0.4 and 0.4±0.2 mV for artificial cerebrospinal fluid (ACSF) and 10 μM ZD7288, respectively, paired t -test P =0.00013, t (3)=25.9, n =4 cells in four slices from two mice) and rebound spiking ( Fig. 6f ). Then we added to the ACSF GABA and glutamate receptor antagonists dl-APV, NBQX, SR-95531 (GBZ), CGP 35348 (referred as antagonist mix). All neurons displayed bursting or regular spiking depending on the imposed membrane potential ( n =15 neurons, Fig. 6g ). VGLUT3 neurons burst frequency ranged from 0.35–6 Hz (ref. 22 ), with a mean of 1.8±1.2 bursts s −1 ( n= 52). We concluded that VGLUT3 neurons were spontaneously active. However, to exclude potential alterations of the firing properties due to the whole-cell configuration, we recorded another set of Vglut3-TOM neurons in cell-attached configuration ( Fig. 6h ). All recorded cells, displayed spontaneous firing persisting after addition of the antagonist mix ( Fig. 6h,i ). On average, the mean firing frequency increased following drug application suggesting that most cells were tonically inhibited ( Fig. 6i ). Moreover, to confirm that VGLUT3/GABAergic neurons were sampled in our recordings, we crossed Vglut3-TOM mice with GAD67-GFP mice and recorded from GFP + /TOM + neurons in presence of the antagonist mix. All GFP + /TOM + cells exhibited similar electrophysiological characteristics ( Fig. 6j–l ) and displayed similar rhythmic activity (burst frequency 1.9±0.2 Hz; n =40 for Vglut3-TOM versus 1.3±0.2 Hz; n= 12 for Vglut3-TOM/GAD67-GFP; Mann–Whitney test, Z (50)=1.3, P =0.2). Taken together, these data suggest that all VGLUT3 neurons, including VGLUT3/GABAergic cells, have similar electrophysiological properties. Finally, it has recently been shown that ET cells can be depolarized by serotonin (5-HT) through direct activation of 5-HT2A receptors [29] . In agreement with this, we found that application of 5-HT increased the spontaneous firing frequency of Vglut3-TOM neurons. The effect was reversed by bath application of the 5-HT2A receptor antagonist 4F-4PP ( Fig. 6m,n ). In another group of cells, we applied the 5-HT2A receptor agonist TCB-2, which increased the spontaneous firing rate in all tested cells ( Fig. 6o ). In summary, despite the heterogeneity observed by immunohistochemistry, all VGLUT3 neurons share similar anatomical and electrophysiological features characterizing ET cells (that is, morphology, spontaneous bursting activity, I h current, response to 5-HT), suggesting that VGLUT3 neurons are ET cells. VGLUT3 neuron response to sensory inputs stimulation ET cells receive monosynaptic inputs from OSNs [4] , [5] , [24] . We thus verified whether VGLUT3 neurons receive direct olfactory nerve (ON) inputs ( Fig. 7a–d ). Low electric stimulation intensity failed to evoke response while higher intensities evoked graded excitatory postsynaptic potential (EPSPs) and bursts of action potentials ( Fig. 7a ) often followed by long-lasting depolarization ( n =8 out of 10 cells; Fig. 7b ). The latency of ON-evoked EPSPs was short ( Fig. 7e ), similar to values reported for monosynaptic ON response in ET cells [4] , [5] , [24] . However, we aimed to confirm that the EPSP latency was compatible with a monosynaptic connection. First, we placed the stimulating electrode above a glomerulus adjacent to the recorded cell. The stimulation-evoked IPSPs were blocked by NBQX and APV, demonstrating the polysynaptic nature of these connections ( Fig. 7c ). The latency of ON-evoked IPSPs was significantly longer than the ON-evoked EPSPs latency ( Fig. 7e ). Second, since D2 and GABA B receptors depress ON synaptic transmission [30] , [31] , [32] , we recorded ON-evoked EPSPs and applied GABA B and D2 receptor agonists (baclofen and apomorphine, respectively; Fig. 7d ). Although the EPSP amplitude decreased ( n =3, from 19±2.2 mV to 5±2.5 mV in control and drugs, respectively; paired t -test, t (2)=8.3, P =0.014), the latency remained unaffected ( Fig. 7e ). Taken together, these data suggest that VGLUT3 neurons receive monosynaptic excitatory inputs from the ON. 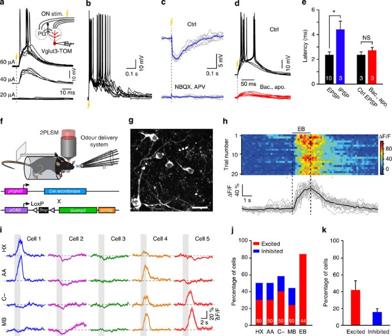Figure 7: Vglut3 neuron responses to sensory inputs stimulation. (a) Synaptic responses evoked by increasing intensities of olfactory nerve (ON) stimulation (20 μA, 40 μA and 60 μA) in a VGLUT3 neuron. Yellow lightning and dotted line indicate ON stimulation (similar convention in subsequent panels). (b) Higher stimulation intensities evoked bursts of APs and long-lasting depolarization. (c) Superimposed traces of ON-evoked IPSPs in another Vglut3-TOM.cell recorded in control and during application of 10 μM NBQX and 100 μM dl-APV. Average traces are shown in blue. (d) ON-evoked response in ACSF (Ctrl) and in the presence of 10 μM (RS)-baclofen and 30 μM apomorphine in a TOM+neuron. (e) Histogram summarizing the latencies of evoked EPSPs and IPSPs for different cells and for different conditions (EPSP versus IPSP: Mann–WhitneyU-test:n=10,Z=−2.28, *P=0.022; Ctrl versus Bac/apo: Wilcoxon matched pairs test:n=3,Z=1.6,P=0.11). White numbers indicate the number of recorded cells. (f) Schema of the experimental procedure: odorant-evoked Ca2+responses were recorded from the somata of Vglut3-GCaMP3 neurons in awake head-restrained mice using a two-photon laser scanning microscope (2PLSM). (g) Z-stack projection of GCaMP3+neurons imaged in an awake mouse (scale bar, 20 μm). (h) Ca2+transients evoked by several repetitions of ethyl butyrate (EB) application imaged in a GCaMP3+neuron. Grey lines: twenty individual trials. Black line: average response. (i) Examples of the averaged Ca2+signals (shaded areas represent s.e.m.) evoked by different odorants in several GCaMP3+neurons. Methyl benzoate (MB), Carvone − (C−), amyl acetate (AA) and 3-Hexanone (HX). Grey boxes indicate odour application. Cells 1–3 and cells 4–5 are representative examples taken from two animals, respectively. (j) Fraction of cells excited and inhibited by different odorants. White numbers indicate the number of imaged cells (n=6 mice). (k) Average fraction of cells excited or inhibited by different odorants. All data are presented as mean±s.e.m. Figure 7: Vglut3 neuron responses to sensory inputs stimulation. ( a ) Synaptic responses evoked by increasing intensities of olfactory nerve (ON) stimulation (20 μA, 40 μA and 60 μA) in a VGLUT3 neuron. Yellow lightning and dotted line indicate ON stimulation (similar convention in subsequent panels). ( b ) Higher stimulation intensities evoked bursts of APs and long-lasting depolarization. ( c ) Superimposed traces of ON-evoked IPSPs in another Vglut3-TOM.cell recorded in control and during application of 10 μM NBQX and 100 μM dl-APV. Average traces are shown in blue. ( d ) ON-evoked response in ACSF (Ctrl) and in the presence of 10 μM (RS)-baclofen and 30 μM apomorphine in a TOM + neuron. ( e ) Histogram summarizing the latencies of evoked EPSPs and IPSPs for different cells and for different conditions (EPSP versus IPSP: Mann–Whitney U -test: n =10, Z =−2.28, * P =0.022; Ctrl versus Bac/apo: Wilcoxon matched pairs test: n =3, Z =1.6, P =0.11). White numbers indicate the number of recorded cells. ( f ) Schema of the experimental procedure: odorant-evoked Ca 2+ responses were recorded from the somata of Vglut3-GCaMP3 neurons in awake head-restrained mice using a two-photon laser scanning microscope (2PLSM). ( g ) Z-stack projection of GCaMP3 + neurons imaged in an awake mouse (scale bar, 20 μm). ( h ) Ca 2+ transients evoked by several repetitions of ethyl butyrate (EB) application imaged in a GCaMP3 + neuron. Grey lines: twenty individual trials. Black line: average response. ( i ) Examples of the averaged Ca 2+ signals (shaded areas represent s.e.m.) evoked by different odorants in several GCaMP3 + neurons. Methyl benzoate (MB), Carvone − (C−), amyl acetate (AA) and 3-Hexanone (HX). Grey boxes indicate odour application. Cells 1–3 and cells 4–5 are representative examples taken from two animals, respectively. ( j ) Fraction of cells excited and inhibited by different odorants. White numbers indicate the number of imaged cells ( n =6 mice). ( k ) Average fraction of cells excited or inhibited by different odorants. All data are presented as mean±s.e.m. Full size image Presently, little is known about the in vivo response of ET cells to odorants. We thus crossed Vglut3-cre mice with a Cre-activated reporter line expressing the genetically encoded Ca 2+ indicator GCaMP3 ( Fig. 7f and Supplementary Fig. 2 ). We monitored fluorescence changes in response to odour applications in individual neurons from awake head-restrained mice ( Fig. 7g–i ). Odorant applications evoked both increase and decrease in fluorescence ( Fig. 7h,i ). The decrease of fluorescence is consistent with a decrease of firing rate mediated by ON-evoked IPSPs ( Fig. 7c ). Depending on the odorant, some cells switched between excitation and inhibition ( Fig. 7i and Supplementary Fig. 2 ). Furthermore, neurons projecting to the same glomerulus had the same odorant-response profile ( Supplementary Fig. 2 ). The fraction of cells excited and inhibited varied across odorants ( Fig. 7j ). On average, odorants excited ~40% of the VGLUT3 cells and inhibited 10% of them ( Fig. 7k ). In summary, VGLUT3 neurons receive direct ON inputs and their odour-evoked response is odorant-specific and tuned by GABAergic neurons. VGLUT3 neurons contact different types of bulbar neurons To identify neurons receiving synaptic inputs from VGLUT3 neurons, we used an optogenetic approach to probe connectivity between Vglut3-ChR2 cells ( Supplementary Fig. 3a–c ) and different populations of OB neurons. Since ET cells are known to directly excite output neurons in the OB [3] , [4] , [5] , we performed whole-cell recordings from these neurons while stimulating Vglut3-ChR2 cells ( Fig. 8a–l ). In some TCs ( n =6), light-evoked EPSPs were recorded at different frequencies of stimulation ( Fig. 8b ). These excitatory connections were small (amplitude of the first EPSP=251±51 μV at 30 Hz light stimulation) but reliable since each action potential of the train evoked an EPSP, suggesting a direct excitatory connection. Consistently, the latency was compatible with monosynaptic connection ( Supplementary Fig. 4 ). In other TCs ( n =2), light stimulation-evoked IPSPs only at high stimulation frequency that were blocked by NBQX/APV and characterized by longer latencies ( Fig. 8c,l and Supplementary Fig. 4 ), suggesting a polysynaptic inhibitory connection. Surprisingly, no PSPs were ever recorded in the mitral cells having intact primary and lateral dendrites at any tested stimulation frequencies, suggesting that VGLUT3 neurons are not the population of ET cells previously reported to excite mitral cells ( Fig. 8d,k ). 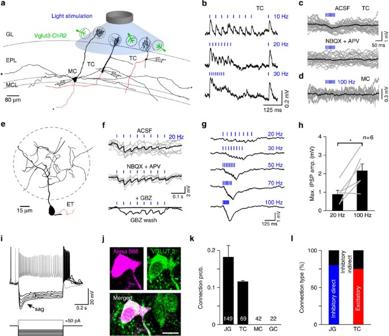Figure 8: VGLUT3 neurons differentially control output neurons of the OB. (a) Schema illustrating the experimental procedure. Montage of different cell types recorded and reconstructed from different slices. MC: mitral cell, TC: tufted cell. Axons appear in red. For simplicity, axons and dendrites were truncated in the illustration (black stars). (b) Light-evoked EPSPs recorded from a TC at different stimulation frequencies. Each trace represents the average of 20 repetitions. (c) Single traces (grey) and average trace (black) showing light-evoked IPSPs recorded from TC in different pharmacological conditions. (d) Single traces (grey) and average trace (black) showing the absence of light-evoked PSP on a representative MC. (e–f) IPSPs evoked by light stimulation in different pharmacological conditions recorded from the VGLUT3-negative ET cell reconstructed in (e). Axon appears in red. (g) Light-evoked IPSPs recorded from a different VGLUT3−ET cell in response to light trains at different frequencies. (h) Histogram showing maximum IPSP amplitude evoked by 20 and 100 Hz light stimulation in VGLUT3−ET cell (Wilcoxon matched pairs test *P=0.046,Z=1.99). Data are presented as mean±s.e.m. (i) Typical response of a VGLUT3−ET cell to injection of negative or positive pulses of current. Note the presence of sag and rebound spiking following hyperpolarization. (j) VGLUT3−ET cell are immunostained for VGLUT2 (scale bar, 10 μm). (k) Graph summarizing the probability of connection made by VGLUT3+neurons onto different cell types of the OB. GC: granule cell. Numbers of recorded cells are indicated on the bars. Error bars are computed assuming binomial distribution (that is, s.e.m.=√[f(1−f)/n], wherefis the fraction of modulated cells andnis the total number of recorded neurons). (l) Graph summarizing the different types of connections recorded from JG cells and TC. Figure 8: VGLUT3 neurons differentially control output neurons of the OB. ( a ) Schema illustrating the experimental procedure. Montage of different cell types recorded and reconstructed from different slices. MC: mitral cell, TC: tufted cell. Axons appear in red. For simplicity, axons and dendrites were truncated in the illustration (black stars). ( b ) Light-evoked EPSPs recorded from a TC at different stimulation frequencies. Each trace represents the average of 20 repetitions. ( c ) Single traces (grey) and average trace (black) showing light-evoked IPSPs recorded from TC in different pharmacological conditions. ( d ) Single traces (grey) and average trace (black) showing the absence of light-evoked PSP on a representative MC. ( e – f ) IPSPs evoked by light stimulation in different pharmacological conditions recorded from the VGLUT3-negative ET cell reconstructed in ( e ). Axon appears in red. ( g ) Light-evoked IPSPs recorded from a different VGLUT3 − ET cell in response to light trains at different frequencies. ( h ) Histogram showing maximum IPSP amplitude evoked by 20 and 100 Hz light stimulation in VGLUT3 − ET cell (Wilcoxon matched pairs test * P =0.046, Z =1.99). Data are presented as mean±s.e.m. ( i ) Typical response of a VGLUT3 − ET cell to injection of negative or positive pulses of current. Note the presence of sag and rebound spiking following hyperpolarization. ( j ) VGLUT3 − ET cell are immunostained for VGLUT2 (scale bar, 10 μm). ( k ) Graph summarizing the probability of connection made by VGLUT3 + neurons onto different cell types of the OB. GC: granule cell. Numbers of recorded cells are indicated on the bars. Error bars are computed assuming binomial distribution (that is, s.e.m.=√[ f (1− f )/ n ], where f is the fraction of modulated cells and n is the total number of recorded neurons). ( l ) Graph summarizing the different types of connections recorded from JG cells and TC. Full size image To determine whether other neuronal populations of the OB would receive synaptic inputs from VGLUT3 neurons, we recorded from granule cells (GCs) but never found responses following light stimulation at any of the tested frequencies ( Fig. 8k ). We also patched JG neurons ( n =149 neurons) including periglomerular (PG) neurons, short-axon cells and neurons displaying an ET cell morphology but being VGLUT3 – . We never found excitatory connections. In contrast, we recorded GABA A -mediated inhibitory connections that were mainly monosynaptic ( n =15/18 connections) since IPSPs were reliably evoked by each action potential at low frequencies and were not blocked by NBQX/APV ( n =15, Fig. 8f ) or a gap junction blocker ( n =3, Supplementary Fig. 5 ). The peak amplitude of light-evoked IPSPs was larger at high frequencies ( Fig. 8g,h ) and the latency was also compatible with a monosynaptic connection ( Supplementary Fig. 4 ). These results are consistent with the immunostaining results, which already suggested that a subpopulation of VGLUT3 neurons expressing GABAergic markers could release GABA ( Figs 2e , 4c and 5d ). Interestingly, all the JG neurons receiving direct inhibitory inputs had the morphology of ET cells, although they were VGLUT3 − ( Fig. 8e ). Interestingly, these VGLUT3 − cells also exhibited electrophysiological properties of ET cells: low input resistance (154±22 MΩ), depolarized resting membrane potentials (−49.2±1.3 mV), presence of a sag and rebound spiking after hyperpolarizing current injection ( Fig. 8i ) and spontaneous firing in ACSF. Besides VGLUT2 labelling confirmed their glutamatergic phenotype ( n =4; Fig. 8j ). To confirm that VGLUT2 + /VGLUT3 − neurons represent a separate population of ET cells, we recorded VGLUT3 − cells in the GL displaying spontaneous rhythmic activity in presence of GABAergic and glutamatergic receptors antagonists. These cells had the morphology and electrophysiological properties of ET cells ( Supplementary Fig. 6a,b ) and all expressed VGLUT2 ( n =7 cells, Supplementary Fig. 6c ). Therefore VGLUT2 is a marker of a different population of ET cells being VGLUT3 − , presumably identifying the previously described ET cells [3] , [4] , [5] , [6] . Taken together, these data suggest that VGLUT3 neurons differentially connect with mitral and TCs. Excitatory connections were never found on mitral cells, but were found on TCs. In addition, VGLUT3 neurons directly inhibited a population of ET cells that are VGLUT2 + but VGLUT3 − . By inhibiting ET cells mediating the multistep excitation, VGLUT3 neurons may affect odour-evoked responses of M/T cells. VGLUT3 neurons suppress the firing of output neurons in vivo We next studied the functional impact of VGLUT3 neurons on the activity of M/T cells in vivo . We used optrodes to record M/T cells [33] , [34] , [35] from control (that is, not expressing channelrhodopsin) and Vglut3-ChR2 mice while stimulating the GL with blue laser ( Fig. 9a,b ). Photostimulation consistently reduced both spontaneous and odour-evoked firing in M/T cells recorded specifically from Vglut3-ChR2 mice ( Fig. 9c–e ). At a population level, a large fraction of M/T neurons were inhibited in Vglut3-ChR2 mice ( Fig. 9f–h ). 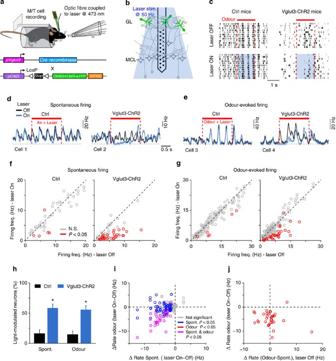Figure 9: VGLUT3 neurons stimulation suppresses the firing of OB output neuronsin vivo. (a,b) Schema illustrating the experimental procedure. Optrodes are placed in the OB to simultaneously record M/T cells and stimulate VGLUT3 neurons expressing channelrhodoposin-2 with a laser-coupled optic fibre. (c) Examples of raster plots for M/T single units recorded in control and in Vglut3-ChR2 mice. Odour-evoked firing is selectively suppressed by photostimulation (laser ON) in Vglut3-ChR2 mice. (d,e) Peristimulus time histogramss) in control (black traces) and during photostimulation (blue traces) show a selective suppression of both spontaneous (d) and odour-evoked (e) firing in M/T cells recorded in Vglut3-ChR2 mice. Shaded areas represent s.e.m. (f,g) Summary plots showing the effect of photostimulation on spontaneous (f;n=42 and 55 single units for ctrl and Vglut3-ChR2 mice, respectively) and odour-evoked (g;n=126 and 165 cell/odour pairs for ctrl and Vglut3-ChR2, respectively) firing. Red circles represent cells displaying a significant rate change evoked by photostimulation (pairedt-testP<0.05 plus Bonferroni correction). (h) Fraction of cells significantly modulated by photostimulation (n=42 and 55 M/T units for ctrl and Vglut3-ChR2, respectively). Error bars are computed assuming binomial distribution (that is, s.e.m.=√[f(1−f)/n], wherefis the fraction of modulated cells andnis the total number of recorded neurons). The fraction of cells modulated by photostimulation is significantly higher in Vglut3-ChR2 mice (χ2test *P=0.0002). (i) Scatter plot showing the effect of photostimulation on both spontaneous and odour-evoked firing for all recorded neurons in Vglut3-ChR2 mice. Each circle represents a cell/odour pair. (j) Scatter plot shows neurons recorded in Vglut3-ChR2 mice and significantly changing their odour-evoked firing after photostimulation. Each circle represents a cell/odour pair. Stimulation suppresses odour-evoked firing independently of whether odour-evoked response in the absence of photostimulation is excitatory or inhibitory. In modulated neurons, the inhibition was strong for both spontaneous and odour-evoked firing (average reduction: 75.7±9% and 61.6±3.4% for spontaneous and odour, respectively) and independent on the basal firing rate ( Fig 9f,g ). Notably, all cells modulated by photostimulation during odour application were also modulated during spontaneous activity ( Fig. 9i ). Finally, the light-evoked suppression of odour-evoked firing was observed in neurons either excited or inhibited by odorants ( Fig. 9j ). Figure 9: VGLUT3 neurons stimulation suppresses the firing of OB output neurons in vivo . ( a , b ) Schema illustrating the experimental procedure. Optrodes are placed in the OB to simultaneously record M/T cells and stimulate VGLUT3 neurons expressing channelrhodoposin-2 with a laser-coupled optic fibre. ( c ) Examples of raster plots for M/T single units recorded in control and in Vglut3-ChR2 mice. Odour-evoked firing is selectively suppressed by photostimulation (laser ON) in Vglut3-ChR2 mice. ( d , e ) Peristimulus time histogramss) in control (black traces) and during photostimulation (blue traces) show a selective suppression of both spontaneous ( d ) and odour-evoked ( e ) firing in M/T cells recorded in Vglut3-ChR2 mice. Shaded areas represent s.e.m. ( f , g ) Summary plots showing the effect of photostimulation on spontaneous ( f ; n =42 and 55 single units for ctrl and Vglut3-ChR2 mice, respectively) and odour-evoked ( g ; n =126 and 165 cell/odour pairs for ctrl and Vglut3-ChR2, respectively) firing. Red circles represent cells displaying a significant rate change evoked by photostimulation (paired t -test P <0.05 plus Bonferroni correction). ( h ) Fraction of cells significantly modulated by photostimulation ( n =42 and 55 M/T units for ctrl and Vglut3-ChR2, respectively). Error bars are computed assuming binomial distribution (that is, s.e.m.=√[ f (1− f )/ n ], where f is the fraction of modulated cells and n is the total number of recorded neurons). The fraction of cells modulated by photostimulation is significantly higher in Vglut3-ChR2 mice ( χ 2 test * P =0.0002). ( i ) Scatter plot showing the effect of photostimulation on both spontaneous and odour-evoked firing for all recorded neurons in Vglut3-ChR2 mice. Each circle represents a cell/odour pair. ( j ) Scatter plot shows neurons recorded in Vglut3-ChR2 mice and significantly changing their odour-evoked firing after photostimulation. Each circle represents a cell/odour pair. Stimulation suppresses odour-evoked firing independently of whether odour-evoked response in the absence of photostimulation is excitatory or inhibitory. Full size image In summary, these data suggest that VGLUT3 neurons can efficiently suppress both basal and odour-evoked firing of M/T cells. In conclusion, by controlling output neurons of the OB, we propose that VGLUT3 neurons reduce the transfer of odorant information to cortical networks. Here we report a previously uncharacterized population of glutamatergic neurons expressing VGLUT3 in the OB ( Figs 1 , 2 , 3 , 4 , 5 ). Using optogenetics, we identified bulbar synaptic targets of VGLUT3 neurons ( Fig. 8 ) and showed that stimulation of VGLUT3 neurons control the transfer of sensory information to cortical structures by suppressing both spontaneous and odour-evoked firing of output neurons ( Fig. 9 ). We used a genetic labelling approach to study the morphological and electrophysiological properties of VGLUT3-expressing neurons in the GL of the mouse OB. Almost all labelled cells in Vglut3-TOM mice expressed VGLUT3 protein suggesting that Vglut3-TOM mice reliably reveal the entire population of VGLUT3 + neurons in the GL ( Fig. 1 ). As reported in several brains regions [36] , [37] , [38] , the expression of VGLUTs in the GL of the OB is developmentally regulated ( Fig. 2 ; Ohmomo et al. [18] ). From our study it emerges that VGLUT3 neurons represent the smallest population of glutamatergic cells in the GL, but its density increases with age. Additional work is required to investigate whether the observed increase in density reflects a switch in VGLUTs expression or an addition of adult-born neurons [39] , [40] , [41] , [42] . Our immunohistochemical characterization suggests that three subpopulations of VGLUT3 neurons can be identified by different markers and soma size: VGLUT1 + /VGLUT3 + , VGLUT2 + /VGLUT3 + and VGAT + /VGLUT3 + ( Figs 2 , 3 , 4 , 5 ). It follows that VGLUT3 neurons can represent three separated subpopulations rather than a single population displaying developmental switching in vesicular transporter expression. In summary, 60% of VGLUT3 + cells are purely glutamatergic (either VGLUT1 + /TOM + or VGLUT2 + /TOM + ) while the remaining VGLUT3 neurons also have a GABAergic phenotype ( Figs 2 , 4 and 5 ). The existence of neurons showing both GABAergic and glutamatergic phenotype, although intriguing, is no longer new. In fact, the three VGLUTs can be expressed by non-glutamatergic neurons such as cholinergic, dopaminergic, noradrenergic, serotoninergic and GABAergic cells (see for review ref. 43 ). In particular, VGLUT3 is expressed by cholinergic neurons in the striatum and GABAergic interneurons in the cortex and hippocampus [13] , [14] , [44] , [45] , [46] , [47] . Co-expression of two vesicular transporters could be used by neurons to co-release neurotransmitters either at the same terminal or at different terminals (see for review ref. 43 ). If expressed on the same vesicle, a synergistic effect may also occur. In this last case, the addition of a vesicular transporter would increase the concentration of the primary neurotransmitter inside synaptic vesicles (see for review ref. 43 ). Future experiments will be needed to determine the precise location of different vesicular transporters within VGLUT3 neurons and the functional relevance of vesicular transporter co-expression. Many authors have described ET cells morphology, basic electrophysiological properties and response to peripheral as well as top-down inputs [22] , [23] , [24] , [25] , [26] , [27] , [28] . The combination of morphological and electrophysiological features uniquely characterizing ET cells was observed for all VGLUT3 neurons, including the GABAergic/VGLUT3 subpopulation. We therefore claim that VGLUT3 neurons are undistinguishable from ET cells. However, the difference between VGLUT3 neurons and formerly identified ET cells relies on their synaptic targets. In the current circuitry model ( Fig. 10a ), although M/T cells receive monosynaptic inputs from OSNs [3] , [4] , [5] , [6] , the excitation may not be sufficient to trigger action potentials [6] . A feedforward (otherwise called multistep) excitatory pathway mediated by ET cells which release glutamate on output neurons is supposed to amplify ON inputs. This mechanism is considered to be particularly important for MCs that receive weaker ON inputs than TCs. By using optogenetics, we found VGLUT3 + neurons exclusively excite TCs but never mitral cells ( Fig. 8 ). This result is not due to inaccurate sampling since we verified that MCs and TCs had intact apical dendrites. Furthermore, we obtained similar results when performing pair recordings of MCs and VGLUT3-TOM neurons (more than 100 pairs were tested and no connections were found). Thus our data indicate that VGLUT3 neurons do not correspond to the population of ET cell previously reported to excite mitral cells [3] , [4] , [5] , [6] . However, we identified another population of cells being VGLUT2 + but VGLUT3 − that also displayed morphological and electrophysiological features of ET cells ( Fig. 8 and Supplementary Fig. 6 ). VGLUT2 + /VGLUT3 − neurons may correspond to the ET cells previously described to excite MCs and mediate the feedforward excitation. Finally, we report a novel subpopulation of ET VGLUT3+ cells directly inhibiting ET VGLUT2+/VGLUT3− cells. 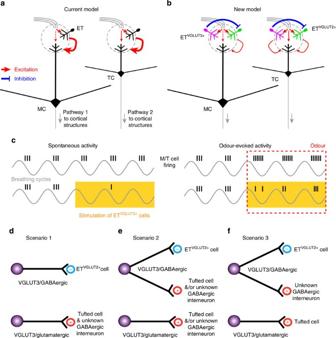Figure 10: Schema summarizing the findings. (a) Current model based on several studies3,4,5,6. Upon nerve stimulation, mitral cells (MCs) receive weak inputs (dotted arrow) from OSNs, and they are mainly stimulated through a multistep excitation mediated by ET cells (thick arrow). Similar mechanism may recruit TCs, although they receive stronger nerve inputs (plain arrow). For clarity, axons from ET cells have been omitted. (b) In the new model, multistep excitation of output neurons would be mediated by ETVGLUT2+/VGLUT3−cells. In addition, we identify a novel population of ETVGLUT3+cells that both excites TCs and inhibits ETVGLUT2+.neurons. When stimulated, VGLUT3+/VGAT+neurons should directly inhibit ETVGLUT2+and reduce the feedforward excitation on M/T cells. It follows that output neurons firing would be reduced. (c) Consistent with the new model, stimulation of VGLUT3+neuronsin vivosuppresses both spontaneous and odour-evoked firing of bulbar output neurons. (d) Possible connectivity patterns involving different VGLUT3 neuron subpopulations. In a first scenario, VGLUT3/GABAergic neurons could specifically contact ETVGLUT2+/VGLUT3−cells while VGLUT3/glutamatergic neurons target TCs. (e) In a second scenario, VGLUT3/GABAergic neurons would release both neurotransmitters at different terminals. The same VGLUT3/GABAergic neuron would inhibit ETVGLUT2+and excite TC and/or unknown GABAergic interneurons. (f) In a third scenario, VGLUT3/GABAergic neurons would release both GABA on ETVGLUT2+and glutamate on GABAergic interneurons that we have not yet identified. In contrast, VGLUT3/glutamatergic neurons would still target TCs. In this scenario, the VGLUT3/GABAergic population would contribute to strongly inhibit output neurons through a complex intra-glomerular inhibition (that is, reduced excitation of output neurons due to inhibition of ETVGLUT2+combined with a feedforward inhibition mediated by excitation of undetermined GABAergic neurons). Figure 10: Schema summarizing the findings. ( a ) Current model based on several studies [3] , [4] , [5] , [6] . Upon nerve stimulation, mitral cells (MCs) receive weak inputs (dotted arrow) from OSNs, and they are mainly stimulated through a multistep excitation mediated by ET cells (thick arrow). Similar mechanism may recruit TCs, although they receive stronger nerve inputs (plain arrow). For clarity, axons from ET cells have been omitted. ( b ) In the new model, multistep excitation of output neurons would be mediated by ET VGLUT2+/VGLUT3− cells. In addition, we identify a novel population of ET VGLUT3+ cells that both excites TCs and inhibits ET VGLUT2+. neurons. When stimulated, VGLUT3 + /VGAT + neurons should directly inhibit ET VGLUT2+ and reduce the feedforward excitation on M/T cells. It follows that output neurons firing would be reduced. ( c ) Consistent with the new model, stimulation of VGLUT3 + neurons in vivo suppresses both spontaneous and odour-evoked firing of bulbar output neurons. ( d ) Possible connectivity patterns involving different VGLUT3 neuron subpopulations. In a first scenario, VGLUT3/GABAergic neurons could specifically contact ET VGLUT2+/VGLUT3− cells while VGLUT3/glutamatergic neurons target TCs. ( e ) In a second scenario, VGLUT3/GABAergic neurons would release both neurotransmitters at different terminals. The same VGLUT3/GABAergic neuron would inhibit ET VGLUT2+ and excite TC and/or unknown GABAergic interneurons. ( f ) In a third scenario, VGLUT3/GABAergic neurons would release both GABA on ET VGLUT2+ and glutamate on GABAergic interneurons that we have not yet identified. In contrast, VGLUT3/glutamatergic neurons would still target TCs. In this scenario, the VGLUT3/GABAergic population would contribute to strongly inhibit output neurons through a complex intra-glomerular inhibition (that is, reduced excitation of output neurons due to inhibition of ET VGLUT2+ combined with a feedforward inhibition mediated by excitation of undetermined GABAergic neurons). Full size image What percentage of ET cells do VGLUT3 neurons represent? If we assume that VGLUT2 is the exclusive marker of ET cells, based on our data reported in Fig. 2d , we can propose that ET VGLUT3 are three times less numerous that ET VGLUT2 . However, there are now evidences that uncharacterized glutamatergic neurons of the GL, which are not ET cells since they display dendrites and axons surrounding the glomeruli [39] , [40] , [41] , [42] , also express VGLUT2. Therefore, the relative fraction of VGLUT3 neurons to the total ET population may be higher than 25%. Taken together, our data suggest that several populations of ET cells are present in the GL and we propose a novel model taking into account this diversity ( Fig. 10b ). In our model, ET VGLUT2+/VGLUT3− neurons would mediate the previously reported feedforward excitation on MCs and TCs. Furthermore, ET VGLUT3+ cells inhibit ET VGLUT2+/VGLUT3− neurons thus reducing the input strength received by M/T cells and consequently their firing rate. Since ET VGLUT3+ cells excite TCs that also receive stronger nerve inputs than MCs [6] , we can speculate that inhibition of the feedforward excitation mediated by ET VGLUT2+/VGLUT3− would affect more MCs than TCs. From our model, VGLUT3 neurons mediate both excitation on TCs and inhibition on ET VGLUT2+ . However, we cannot say whether different subpopulations (that is, VGLUT3/GABAergic versus VGLUT3/purely glutamatergic) would contact ET VGLUT2+ and TCs or if the same subpopulation (that is, VGLUT3/GABAergic) mediates both effects ( Fig. 10a–c ). In addition, stimulation of VGLUT3 cells evoked polysynaptic inhibition on TCs and on ET VGLUT2+/VGLUT3− . We have not yet been able to identify the GABAergic interneurons excited by VGLUT3 neurons that are responsible for this polysynaptic inhibition since granule and periglomerular cells failed to show light-evoked excitation. However, given that each of these interneuron populations is thought to be extremely heterogeneous, we cannot rule out that subpopulations of granule or periglomerular cells, not sampled in our recordings, would receive direct excitation from VGLUT3 neurons. Furthermore, short-axons cells or parvalbumin interneurons in the EPL [48] , [49] , which were not sampled in our recordings, may account for the polysynaptic inhibition. Future studies will be needed to characterize the connectivity of specific VGLUT3 subpopulations as well as the precise origin of the synaptic contacts onto targeted neurons (axonal versus dendritic). Our in vitro data suggested that VGLUT3 neurons might control M/T cells firing. In agreement, VGLUT3 neuron stimulation strongly suppresses both spontaneous and odour-evoked firing in a large fraction of M/T cells in vivo , although some cells were unaffected ( Figs 8 , 9c ). This non-homogenous effect is likely to be due to the local nature of the photostimulation when using optrodes. However, weakly modulated neurons may also represent heterogeneity of response in the M/T cell population. Based on our in vitro data, we can speculate that MCs and TCs may be differentially modulated in vivo . MCs discharge following sensory inputs stimulation is more dependent on multistep excitation than TCs [6] . Therefore, inhibition of ET VGLUT2+ by ET VGLUT3+ could have a more prominent impact on MCs than on TCs. Given that MCs and TCs are not discharging in the same phase in the respiratory cycle [50] and that they project to different cortical structures [51] , modulation by VGLUT3 neurons could differentially control the two output pathways of the OB. By controlling OB output neurons VGLUT3 cells contribute to control the transfer of information from sensory neurons to cortical centres and therefore participate in filtering out odorant information. But how are VGLUT3 cells going to be activated? A first way to recruit VGLUT3 neurons would be through direct synaptic inputs coming from OSNs. VGLUT3 neurons are also strongly inhibited either spontaneously or when the olfactory nerve is stimulated. Combination of excitation and inhibition will lead to complex odorant-specific recruitment of VGLUT3 neurons, as observed in calcium-imaging experiments ( Fig. 7 ). A second way to activate VGLUT3 neurons would be through activation of serotoninergic afferents. We show that VGLUT3 neurons can be depolarized by 5-HT through activation of 5-HT2A receptors. Excitation of all VGLUT3 neurons through 5-HT-2A receptors would be part of a general mechanism of control of input/output gain mediated by 5-HT, decreasing the release of glutamate by sensory neurons [52] and weakening the feedforward excitation pathway. In conclusion, we propose that VGLUT3 neurons represent a novel population of bulbar neurons ideally positioned to control the transfer of odorant information from sensory neurons to cortex while being under the control of both bottom-up and top-down inputs. Animals Tg(Slc17a8-icre) 1Edw mice (referred as Vglut3-cre mice in the text, (ref. 53 )) were crossed with three different Cre-activated reporter lines conditionally expressing either tdTomato [54] , Channelrhodopsin2-YFP [55] or GCaMP3 (ref. 56) [56] . We analysed the progeny derived from these crossings carrying the Cre driver and one reporter allele (referred as Vglut3-TOM, Vglut3-ChR2 and Vglut3-GCaMP3 mice in the text). In few experiments, Vglut3-cre::Rosa-floxStopflox-tdTom mice were crossed with GAD67-GFP knock-in mouse Gad1 tm1Tama (ref. 57 ). C57BL/6J mice were also used for data presented in Figs 4 and 9 . None of the experiments were performed blind of the genotype. Animals used for the experiments were coming from different litters. Both genders have been used throughout the study. Mice age is reported in other method sections or in figure legends. All animal protocols are in accordance with the Swiss Federal Act on Animal Protection, Swiss Animal Protection Ordinance and were approved by the University of Geneva and Geneva state ethics committees (authorizations 1007/3387/2 and 1007/3758/2). Immunohistochemistry Animals of different ages (see below and results) were deeply anaesthetized with an intraperitoneal injection of urethane 20% in 0.9% NaCl and perfused transcardially with 40 ml of saline followed by 50 ml of 4% paraformaldehyde (PFA) in 0.1 M phosphate buffer at 4 °C (phosphate-buffered saline (PBS), pH 7.3). The brains were then dissected out and postfixed overnight in 4% PFA. After embedding brains in 4% agarose, 40 μm slices (either coronal or horizontal) were cut with a vibratome (Leica VT S1000) and collected in PBS (0.1 M). To stain YFP + neurons, we first blocked endogenous peroxidases by incubating the sections for 20 min with 0.7% H 2 O 2 in TBSTT (Tris-buffered saline with tween and triton). After rinsing, they were blocked with 10% normal goat serum for 1 h at room temperature and then incubated with rabbit anti-GFP antibody overnight at 4 °C (1:1,000, Invitrogen). The day after, slices were rinsed and incubated with biotinylated goat anti-rabbit IgG (1:200, Invitrogen, catalogue number A11122) for 1 h at room temperature. Sections were then processed using avidin–biotin–peroxidase complex (ABC kit, Vector Laboratories) and reacted with the chromogen 3,3′ diaminobenzidine (DAB, Sigma-Aldrich). Sections were mounted with DePeX mounting medium (Gurr). For the age-dependent expression analysis, we used 2-, 4- and 8-week-old Vglut3-Tom mice ( n =4 animals in each group). For each staining, at least 100 cells (imaged from ~40 stacks taken from ~6 different slices) were analysed per animal. Slices were incubated with one or two primary antibodies overnight, followed by appropriate secondary antibodies. Primary antibodies used were: rabbit anti-VGLUT1 (1:2,000, Synaptic Systems, cat. num. 13530); rabbit anti-VGLUT2 (1:1,000, Synaptic Systems, cat. num. 135403), rabbit anti-VGLUT3 (1:1,000, Synaptic Systems, cat. num. 135203); rabbit anti-VGAT (1:400, Synaptic Systems, cat. num. 131003); mouse anti-GAD67 (1:1,000, Millipore; cat. num. MAB5406), rabbit anti-Calretinin (1:1,000, Swant, cat. num. 7699/4); rabbit anti-Calbindin (1:500, Swant, cat. num. 300); mouse anti-TH (1:500, Chemicon, cat. num. MAB5280). Secondary antibodies used were: Alexa 488 anti-rabbit (Invitrogen, cat. num. A21206), Alexa 546 anti-mouse (Invitrogen, cat. num. A21123), Alexa 647 anti-mouse (Invitrogen, cat. num. A31571). All secondary antibodies were diluted 1:200. Slices were counterstained with Hoechst (1:5,000, Invitrogen, cat. num. H3570) and mounted with Vectashield (Vector Laboratories). Images were acquired with a confocal laser scanning microscope (Zeiss LSM 700) with × 63 oil-immersion objective. Fluorescent channels were acquired in sequence to separate wavelength and minimize possible cross-talk. Projection images were made in ImageJ. Quantification of co-localization was done with the Zeiss LSM browser. Slice electrophysiology Experiments were performed on 6–8-week-old Vglut3 -Tom or Vglut3 -ChR2 mice. Animals were anesthetized by isoflurane inhalation before decapitation. OB extraction and dissection were done as previously described [58] , [59] . In brief, horizontal slices (thickness=300 μm) were cut with a vibratome (Leica VT S1000) in ice-cold cutting solution containing (in mM): 83 NaCl, 2.5 KCl, 0.5 CaCl 2 , 3.3 MgSO 4 , 26.2 NaHCO 3 , 1 NaH 2 PO 4 , 22 D -glucose and 72 sucrose. Slices were transferred to normal ACSF at ~34 °C for 30 min and then stored at room temperature before the experiment. The normal ACSF used during recordings contained (in mM): 124 NaCl, 3 KCl, 2 CaCl 2 , 1.3 MgSO 4 , 26 NaHCO 3 , 1.25 NaH 2 PO 4 , 10 D -glucose with osmolarity of 300 mOsm and pH=7.4 when bubbled with 95% O 2 -5% CO 2 . Individual slices were transferred to the recording chamber and perfused with oxygenated ACSF. All recordings were performed at 37 °C (±0.5 °C). Whole-cell and cell-attached recordings were performed using an IR-DIC microscope (Olympus BX51). Recordings were performed using borosilicate glass pipettes with resistance of 4–8 MΩ and filled with an intracellular solution (mM) containing: 110 K-gluconate, 10 KCl, 10 HEPES, 4 ATP, 0.3 GTP, 10 phosphocreatine and 0.4% biocytin and pH between 7.2 and 7.3. Recordings were amplified using Multiclamp 700A amplifiers (Molecular Devices, USA), filtered at 4 KHz, digitized (5–20 KHz) and acquired using PulseQ electrophysiology package running on Igor Pro (Wavemetrics, USA). ON stimulation was achieved using a bipolar electrode. The ON was identified under DIC and the electrode was placed on the nerve, in the vicinity of the glomerulus in which the VGLUT3 neuron projected its apical dendrite. The electrical stimuli (200 μs) were delivered at 0.33 Hz using an isolated pulse stimulator (A-M Systems). For optogenetic experiments, we stimulated Vglut3-ChR2 neurons with a LED (Thorlabs, Germany, 2–10 ms pulses) replacing the halogen light source transmission of the microscope. All recorded neurons kept for the connectivity analysis had intact dendritic arborizations (for example, intact primary and secondary dendrites for M/T cells). The power after the objective was set to 0.6–0.8 mW × mm 2 and maintained constant during the experiments. The objective (Olympus, LUMPLFLN 40XW, numerical aperture=0.8 and working distance=3.33 mm) was positioned either on top of the GL, EPL or GC layer (different locations have been tested during the recordings of the same cell). During photobleaching experiments (light on for an hour), we estimated that the bleached area had a diameter of ~300–400 μm. However, during the short pulse of light illumination (2–10 ms), the area efficiently recruiting ChR2-expressing cells may be smaller. 2,3-dioxo-6-nitro-1,2,3,4-tetrahydrobenzo[ f ]quinoxaline-7-sulphonamide disodium salt (NBQX), DL-2-amino-5-phosphonovaleric acid (APV), SR-95531 (gabazine), (3-aminopropyl)(diethoxymethyl)phosphinic acid (CGP 35348), 5-HT hydrochloride (5-HT), 4-(4-fluorobenzoyl)-1-(4-phenylbutyl) piperidine oxalate (4F-4PP), (4-Bromo-3,6-dimethoxybenzocyclobuten-1-yl) methylamine hydrobromide (TCB-2), (RS)-Baclofen and ZD7288 were purchased from Tocris (Bristol, UK). All salts and (R)-(-)-Apomorphine hydrochloride was purchased from Sigma-Aldrich (Germany). Data processing and analysis were done using Igor (Wavemetrics), Matlab (Mathworks) and Excel (Microsoft Office). Data are reported as mean±s.e.m. To confirm the identity of recorded neurons, either 1 mM Alexa 488 hydrazide or 1 mM Alexa 568 hydrazide (Invitrogen) was included in the intracellular solution. Biocytin staining was used to analyse neuron morphology. Briefly, slices were fixed for 3 h in phosphate buffer (pH 7.4) containing 4% PAF. Thereafter, slices were transferred into phosphate-buffered saline (PBS) containing 3% H 2 O 2 to block endogenous peroxidases. After rinsing, slices were incubated for 2 h with avidin–biotin complex. The samples were then rinsed again and developed with diaminobenzidine under bright field microscope until the cells were visible. The reaction was stopped transferring the slices in PBS. Finally, slices were mounted on slides using 85% glycerol. Cells were reconstructed in bright field under a × 100/1.30 NA oil-immersion objective using Neurolucida system (MicroBrightField). Some slices containing JG neurons receiving direct inhibitory connection from Vglut3-ChR2 cells were fixed in 4% PAF as describe above and immunostaining for VGLUT2 (1:1,000, Synaptic Systems, cat. num. 135403) was performed in 300 μm slices. Slices were incubated with TBSTT at least for 6 h to maximize antibodies penetration. Odorants and stimulation The odorants used were methyl benzoate (MB, ≥98% purity), amyl acetate (AA, ≥99%), ethyl butyrate (EB, ≥99%), Carvone −(C−, >95%), 3-Hexanone (Hx, ≥98% purity). All chemicals were obtained from Sigma-Aldrich or Fluka Chemie (Steinheim, Germany). Odorants were delivered through a custom made olfactometer during an animal’s expiration as described previously [34] , [60] . The air flow passed through the vials containing the odorants. The total flow was constant (0.4 l min −1 ). To maintain a stable odour concentration during the entire stimulus application, we ensured that flows were stationary with a 5-s preloading before the odorant was delivered. 2-photon calcium imaging Three-to-four month-old Vglut3-GCaMP3 mice were anesthetized with an intraperitoneal injection of a mixture of midazolam (0.4 mg kg −1 ), medetomidine (2 mg kg −1 ) and fentanyl (100 μg kg −1 ). By placing the mouse on a custom made heating pad, we monitored body temperature. Animals were implanted with a stainless steel headpost that was firmly attached to the skull with dental cement (Syntac Assortment, Ivoclar Vivadent Clinical, Liechtenstien). A cranial window of 2.5 mm diameter was then drilled on the central part of the OB in order to avoid damages to the blood vessels located under caudal part of the bone that overlay the structure. A 3 mm cover glass was then sealed on top of the craniotomy with dental cement. To reverse the anesthesia, animals were injected subcutaneously with a mixture of flumazenil (4 mg kg −1 ), naloxone (0.8 mg kg −1 ) and atipamezole (20 mg kg −1 ). All mice were allowed to recover for 7 days after surgery and then trained for 7 days to be head restrained. To perform calcium imaging in awake mice, we used a × 20 Olympus objective (0.95 NA) mounted on a custom made microscope controlled with ScanImage [61] ( http://www.scanimage.org ). GCaMP3 was excited using a Ti-Sapphire laser (Chameleon ultra II, Coherent) tuned to λ =910 nm. The field of view was 200 × 200 μm and images were acquired at a resolution of 512 × 128 and a frequency of 7.81 Hz. The imaging protocol consisted of a series of 20 trials corresponding to 20 successive odour applications. The breathing cycle was monitored during imaging sessions and used to synchronize odour application onset to the end of animals’ inspiration via a slope/height window discriminator (FHC, Bowdoinham, USA). Each trial lasted ~17 s with 5-s odour preloading (odorant stream bypassing the animal), a 200-ms delay period during which the breathing cycle could trigger odour delivery, a 2-s odour application and a 10-s post odour period. Images were analysed offline using ImageJ and custom analysis routine written in Matlab. Briefly, circular regions of interest were placed on GCaMP3-expressing cells to extract their changes in fluorescence intensity over time. For each ROI, the change in fluorescence relative to baseline (ΔF/F) was calculated and filtered with a 3-point moving average filter. A cell was considered responsive when a Ca 2+ change was detected in more than 10 trials out of 20 and within a time window 0–2 s after odour onset. We set a threshold for detecting evoked Ca 2+ responses as 2 σ , where σ is the s.d. calculated over 5-s baseline activity before odour onset. Statistical analysis In this study, we used analys of variance ANOVA and post hoc test, two-tailed paired and unpaired t -test, χ 2 test and different non-parametric tests (see text and legends). Shapiro–Wilk test was used to assess normality of the data. For all parametric ANOVA, homogeneity of variance was tested using Levene’s test or a test of sphericity (for one-way repeated measures ANOVA). No animal, cell or outlier has been excluded from the data set. In vivo electrophysiology The initial animal preparation, recording procedure and spike sorting analysis have been extensively presented elsewhere [33] , [34] , [62] . For all experiments, respiration was monitored using a directional air flow sensor (AWM2100V, Honeywell, MN) placed in front of the mouse snout. This sensor did not occlude the mouse nose and indeed did not stop the odour from reaching the nostrils. Three month-old Vglut3-ChR2 and C57Bl6J mice were anesthetized with an intraperitoneal injection of a mixture of midazolam (0.4 mg kg −1 ), medetomidine (2 mg kg −1 ) and fentanyl (100 μg kg −1 ). A 1–2 mm window was drilled above the OB and the dura mater was opened. One silicon-based recording optrode (A1 × 32-Poly3-5mm-50s-177-OA32, NeuroNexus Technologies, Ann Arbor, MI, USA) was inserted. Photostimulation was done by connecting the optrode to a fibre-coupled blue laser (SDL-473-050MFL, Shangai dreamlasers, Shangai, China). For all recordings, the laser power was set such that the power at the end of the fibre connected to the laser head was 20 mW. Photostimulation consisted of a train of 60 light pulses (10-ms pulse, 50 Hz) synchronized to odour onset. The skull cavity was filled with an ophthalmic gel (Lacryvisc, Alcon) to protect the brain from drying. A silver wire contacting the gel was connected to the air table to ground the preparation. Electrodes were lowered vertically in the target zone until the mitral/tufted cell layer was reached. It must be noted that our recording electrodes had low impedances (1–4 MΩ at 1 kHz). Stability and reasonable size of the extracellular spike with respect to background noise are two necessary conditions for single-cell identification (clustering, see below), which in the case of low impedance electrodes could only be fulfilled by mitral and TCs (the larger cells in the OB), as observed by others [33] , [35] , [63] , [64] , [65] , [66] . Further details about recording and spike sorting have been described extensively elsewhere [33] , [34] . In brief, wide-band field potentials were amplified ( × 100) and band-pass filtered (0.1 Hz to 9 kHz). All data were digitized at 32,556 Hz with the Cheetah Digital Lynx system (Neuralynx, Tucson, AZ). Spikes were detected by a threshold on the high-pass filtered signal, decomposed in 16 features and automatically clustered by the KlustaKwick software [67] . Obtained clusters were manually merged in Klusters software [68] when they showed a clear refractory period in the cross-correlation of their spike trains. Individual neurons were finally identified as the clusters showing a clean refractory period in their autocorrelation. All subsequent analyses and statistics were calculated using custom scripts written for Matlab (MathWorks, Natick, MA). Fifteen trials for each condition (eight conditions: spontaneous and three odorants tested with and without photostimulation) have been used. All trials for different conditions have been presented randomly. To characterize the effect of photostimulation, we calculated each cell’s firing during spontaneous and odour application by computing the average firing rate on the first two breathing cycles following stimulus onset (for spontaneous firing, no odour was applied). We compared the firing rate with and without photostimulation using the sign test. How to cite this article : Tatti, R. et al. A population of glomerular glutamatergic neurons controls sensory information transfer in the mouse olfactory bulb. Nat. Commun. 5:3791 doi: 10.1038/ncomms4791 (2014).